Turnover time of fluorescent dissolved organic matter in the dark global ocean Marine dissolved organic matter (DOM) is one of the largest reservoirs of reduced carbon on Earth. In the dark ocean (>200 m), most of this carbon is refractory DOM. This refractory DOM, largely produced during microbial mineralization of organic matter, includes humic-like substances generated in situ and detectable by fluorescence spectroscopy. Here we show two ubiquitous humic-like fluorophores with turnover times of 435±41 and 610±55 years, which persist significantly longer than the ~350 years that the dark global ocean takes to renew. In parallel, decay of a tyrosine-like fluorophore with a turnover time of 379±103 years is also detected. We propose the use of DOM fluorescence to study the cycling of resistant DOM that is preserved at centennial timescales and could represent a mechanism of carbon sequestration (humic-like fraction) and the decaying DOM injected into the dark global ocean, where it decreases at centennial timescales (tyrosine-like fraction). The biological pump has long been recognized as a mechanism to remove CO 2 from the atmosphere, through photosynthesis and export of particulate and dissolved organic matter (DOM) to the deep ocean [1] . More recently, the transformation of biologically labile organic matter into refractory (long lifetime in the dark ocean) [2] compounds by prokaryotic activity has been termed the ‘microbial carbon pump’ and may also constitute an effective mechanism to accumulate reduced carbon in the dark ocean [3] , [4] . Given the large pool of refractory DOM (RDOM) in the oceans (~656 pg C) [2] , understanding its generation, transformation and role in carbon sequestration is crucial in regards to understanding present and future CO 2 emission scenarios. Some components of the marine RDOM pool absorb light and a fraction of them also emit fluorescence (fluorescent DOM, FDOM) [5] , [6] . These optical properties are used as tracers for circulation and biogeochemical processes in the dark ocean [7] . Here we obtain the distribution of FDOM in the ocean interior by measuring fluorescence intensities scanned over a range of excitation/emission wavelengths during the Spanish Malaspina 2010 circumnavigation of the globe ( Fig. 1 ). Discrete fluorescent fractions can be discriminated from the measured spectra by applying parallel factor analysis (PARAFAC) [8] (see Methods). Four fluorescent components are isolated from the whole data set and appear to be ubiquitous and common in the dark global ocean [5] , [6] . Two components (C1 and C2) have a broad excitation and emission spectra, with excitation and emission maxima in the ultraviolet and visible region, respectively. These are traditionally referred to as humic-like components, which accumulate and have turnover times of 435±41 and 610±55 years, respectively. These turnover times are longer than the ~350 years that the dark (>200 m) global ocean takes to renew [9] . The two other components (C3 and C4) have narrower spectra with excitation and emission maxima below 350 nm and are similar to the spectra of tryptophan and tyrosine, respectively [10] . The dark global ocean appears to be a sink for fluorescent tyrosine-like (C4) component and has a turnover time of 379±103 years that is comparable to turnover time of DOC pool (estimated in 370 years [11] ). Thus, we propose that the fluorescent fractions of DOM are suitable proxies for determining the cycling of the RDOM that produces (humic-like) and decays (tyrosine-like) in the dark ocean at centennial timescales. 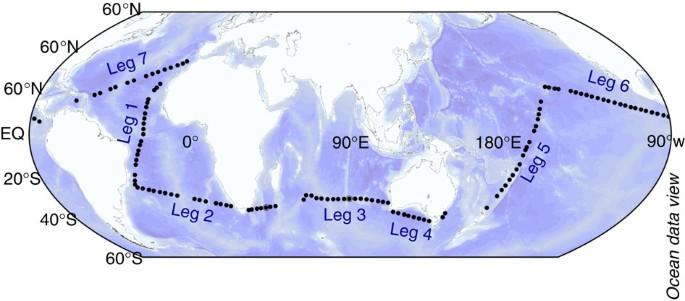Figure 1: Cruise track of the Malaspina 2010 circumnavigation. The cruise departed from Cartagena (Spain) on 17 December 2010 and returned to the same port on 15 July 2011, and was divided into seven legs. Figure 1: Cruise track of the Malaspina 2010 circumnavigation. The cruise departed from Cartagena (Spain) on 17 December 2010 and returned to the same port on 15 July 2011, and was divided into seven legs. Full size image Water masses across the circumnavigation The water mass composition of each water sample was described through the mixing of prescribed water types (WT) with a multi-parameter analysis (see Methods). We identified 22 WT (see Table 1 ) with 12 of them representing 90% of the total volume of water samples collected during the global cruise ( Fig. 2 ). Circumpolar Deep Water (CDW) was widely distributed in the Indian and Pacific Oceans accounting for up to 25.6% of the total volume sampled. North Atlantic Deep Water of 2.0 °C (NADW 2.0 ) and 4.6 °C (NADW 4.6 ) accounted 21.4% of the total volume and mostly located in the Atlantic basin; Antarctic Intermediate Water of 3.1 °C (AAIW 3.1 ) and 5.0 °C (AAIW 5.0 ) accounted for 7.6% of the total volume and spread out through the South Atlantic and Indian basins; and North Pacific Intermediate Water accounted for 5.7% of the total volume sampled. Table 1 Archetypal values of the depth ( Z i ), AOU (AOUi) and the four fluorescent components ( F max1i, F max2i, F max3i and F max4i) for the different WTs intercepted during the Malaspina 2010 circumnavigation. 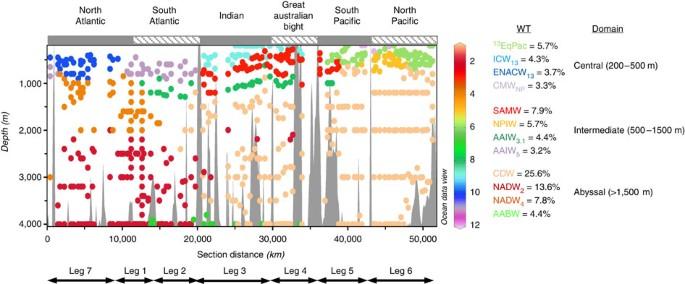Figure 2: Proportions of the main WT intercepted during Malaspina 2010. The percentages represent the proportion of the total volume of water sampled during the cruise that corresponds to each WT. Here the 12 most abundant WT are presented. Note that the depth range starts at 200 m. For more details seeTable 1. Full size table Figure 2: Proportions of the main WT intercepted during Malaspina 2010. The percentages represent the proportion of the total volume of water sampled during the cruise that corresponds to each WT. Here the 12 most abundant WT are presented. Note that the depth range starts at 200 m. For more details see Table 1 . Full size image Global distribution of fluorescent components The maximum fluorescence intensity ( F max) of the two humic-like components (C1 and C2) obtained during the Malaspina circumnavigation showed a global distribution similar to the apparent oxygen utilization (AOU; Fig. 3a–c ), reaching their maxima in the Eastern North Pacific central and intermediate waters and their minima in the Indian Ocean central waters. In contrast, this global trend with AOU was not evident for the two amino-acid-like components (C3 and C4; Fig. 3d,e ). 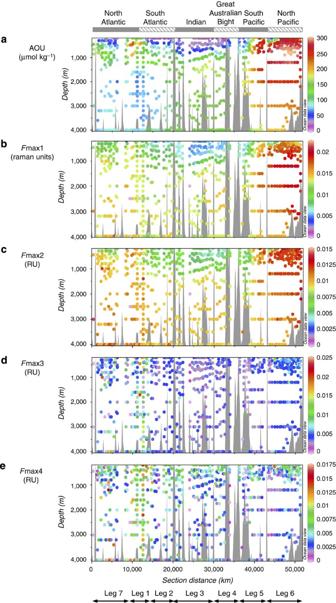Figure 3: Global distribution of the AOU and fluorescence components. The AOU (a) and the fluorescence intensity at the excitation–emission maxima of each component (Fmax) of the four components (b–e) discriminated by the PARAFAC analysis in the global ocean data set of the Malaspina 2010 Expedition are plotted. Note that the depth range starts at 200 m. See Methods andSupplementary Fig. 2for a detailed description of the four fluorescence components. Figure 3: Global distribution of the AOU and fluorescence components. The AOU ( a ) and the fluorescence intensity at the excitation–emission maxima of each component ( F max) of the four components ( b – e ) discriminated by the PARAFAC analysis in the global ocean data set of the Malaspina 2010 Expedition are plotted. Note that the depth range starts at 200 m. See Methods and Supplementary Fig. 2 for a detailed description of the four fluorescence components. Full size image Relationships between the archetypal AOU and fluorophores Combining the outputs from the water mass, AOU and fluorescence analyses, we calculated WT proportion-weighted average values, hereafter referred to as archetypal, for the AOU and the fluorescence intensities of the four components (see Methods). Archetypal values retain the variability associated with the initial concentrations at the site where each WT is defined and its transformation by basin-scale mineralization processes up to the study site [12] . Archetypal concentrations explained 81, 77, 75, 24 and 26% of the total variability of AOU, C1, C2, C3 and C4, respectively ( Table 1 ). In Fig. 4 , we show the measured maximum fluorescence intensity (grey dots), archetypal values for each WT (white dots) and archetypal values for each sample (black dots) for the components C1, C2, C3 and C4 ( Fig. 4a–d , respectively). We obtained direct relationships between the archetypal humic-like components (C1 and C2) and archetypal AOU ( Fig. 4a,b ) suggesting a net production of these components in parallel with the water mass ageing. The relatively high archetypal fluorescence of C1 (blue dots in Fig. 4a ) for North Atlantic Deep Water (NADW) is related to the high load of terrestrial fluorescent materials transported by the Arctic [6] , [13] , [14] rivers, whereas the cause of the high value for the Mediterranean water (MW) is due to the low proportion of this water mass (9±14%) compared to the proportion of NADW (76±33%) in the same sample. Therefore, it is expectable that the archetypal concentration of C1 that our data set produces for the MW should be close to the NADW archetype. For C2, the North Pacific Subtropical Mode Water (STMW NP ; green dot in Fig. 4b ) also departed from the general archetypal C2–AOU trend. Archetypal C1 and C2 can be modelled with archetypal AOU values using power functions ( Fig. 4a,b ). Given that the high fluorescence of NADW and MW in C1 and of STMW NP in C2 is not related to ageing, these water masses were excluded from their corresponding regression models. It is noticeable that the power factor for C1 (0.51±0.04) is almost twice than for C2 (0.31±0.04), indicating a higher C1 production rate per unit of consumed oxygen. Furthermore, in hypoxic waters (dissolved oxygen concentrations <60 μM (ref. 15 ); orange dots in Fig. 4a,b ), C1 and C2 also behave differently; whereas C1 production was enhanced, C2 did not change substantially. 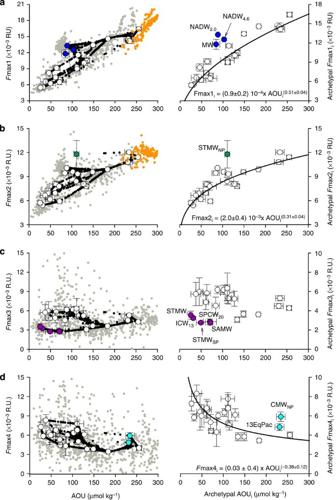Figure 4: Relationships between the fluorescence components and the AOU. Measured concentrations (grey dots), archetypal concentrations for each WT (white dots) and archetypal concentrations for each sample (black dots) for the components C1 (a), C2 (b), C3 (c) and C4 (d). Orange dots represent hypoxic samples. In the right column are presented the regression models and fitting equations for the archetypal values of C1 (R2=0.90,P<0.001,n=19), C2 (R2=0.79,P<0.001,n=21) and C4 (R2=0.31,P<0.05,n=20) with AOUi. WT shown in blue, green and cyan dots were excluded from their respective regression models. Error bars represent the s.d. of the estimated archetypal values of AOU and the four fluorescent components for each WT (see Methods; equation (6)). Figure 4: Relationships between the fluorescence components and the AOU. Measured concentrations (grey dots), archetypal concentrations for each WT (white dots) and archetypal concentrations for each sample (black dots) for the components C1 ( a ), C2 ( b ), C3 ( c ) and C4 ( d ). Orange dots represent hypoxic samples. In the right column are presented the regression models and fitting equations for the archetypal values of C1 ( R 2 =0.90, P <0.001, n =19), C2 ( R 2 =0.79, P <0.001, n =21) and C4 ( R 2 =0.31, P <0.05, n =20) with AOUi. WT shown in blue, green and cyan dots were excluded from their respective regression models. Error bars represent the s.d. of the estimated archetypal values of AOU and the four fluorescent components for each WT (see Methods; equation (6)). Full size image In contrast, we do not observe a significant relationship between the archetypal values of the tryptophan-like fluorescence component (C3) and AOU ( R 2 =0.001, n =22, P =0.88; Fig. 4c ). This lack of correlation is caused by the low archetypal fluorescence (<4 × 10 −3 RU) of the relatively young (AOU<75 μmol kg −1 ) central waters of the Indian and South Pacific oceans (ICW 13 , STMW I , SAMW, SPCW 20 and STMW SP ; Table 1 ; purple dots in Fig. 4c ). However, such low archetypal values are not observed in the tyrosine-like component (C4), leading to a weak but significant inverse power relationship with AOU ( Fig. 4d ). The archetypal tyrosine-like fluorescence of the aged Central waters (AOU>200 μmol kg −1 ) of the Equatorial (13EqPac) and Central North Pacific (CMW NP ) exceeded the expected value from their AOU (cyan dots in Fig. 4d ). These two WT were excluded from the regression model. Net FDOM production and turnover times On the basis of the relationships observed between the archetypal fluorescence intensity of three out of four fluorescence components (C1, C2 and C4) and AOU, we calculated the net production rate of each component, termed net FDOM production (NFP). A positive value of NFP indicates net production, as for the case of the humic-like components C1 and C2, and a negative value indicates net decay, as for the case of the amino-acid-like C4. The NFP of each component was calculated by multiplying the WT proportion-weighted average fluorescence production values per unit of AOU by the oxygen consumption rate (OCR) for the dark ocean (see Methods). Here we have used a conservative OCR estimate of 0.827 pmol O 2 per year [16] . The net humic-like fluorescence production rate obtained was 2.8±0.2 × 10 −5 Raman units per year (RU per year) for C1 and 1.5±0.1 × 10 –6 RU per year for C2, whereas C4 was consumed at a net rate of −1.3±0.2 × 10 −5 RU per year in the dark global ocean. Turnover times of components C1, C2 and C4 were calculated dividing the WT weighted-average fluorescence values of the dark global ocean by its corresponding NFP rate (see Methods). These values represent the time required to produce (C1, C2) or consume (C4) a fluorescence signal of the same intensity than the actual fluorescence of the dark ocean. The resulting turnover of C2, 610±55 years, was significantly longer than the turnover of C1, 435±41 years, and both exceeded the turnover times of the bulk DOC pool—estimated in 370 years [11] —and the terrestrial DOC in the open ocean—estimated in <100 years [17] —as well as the renewal time of the dark ocean (water depths >200 m)—estimated in 345 years [9] . Conversely, the turnover time of the tyrosine-like component C4 in 379±103 years was compatible with the turnover time of the bulk DOC. The global pattern in the dark ocean of an increase in the humic-like components concomitant to water mass ageing (high AOU values) has been previously reported [5] , [6] , [18] , [19] . Although it has been recently hypothesized that this relationship could also be caused by further transformations of terrestrial humic-like materials in the open ocean [20] , culture experiments have unequivocally demonstrated that these materials can be produced in situ in the oceans [21] . In fact, we observe positive and significant relationships between the archetypes of both humic-like components (C1 and C2) and the AOU ( Fig. 4a,b ). The higher C1 production rate per unit of consumed oxygen in comparison with C2 could be related to different mechanisms of production [6] that might be linked to the phylogenetic nature of producers (bacteria, archaea or eukarya) [22] and/or the sensitivity to environmental oxygen concentration. The particularly high archetypal fluorescence of C1 for North Atlantic Deep Water (NADW) has been previously described and appears to be clearly related to the high load of FDOM of terrestrial origin transported from the Arctic rivers to the North Atlantic Ocean [6] , [13] , [14] with a relevant proportion of unaltered high molecular weight lignin [23] . However, the cause of the high C2 signature for the North Pacific Subtropical Mode Water has not been previously reported. We hypothesize that it could be related to intense rainfall south of the Kuroshio extension where these water mass is formed [24] , since it is known that rainwater is particularly enriched in these fluorescent compounds [25] , [26] and this WT is very shallow (archetypal depth=277±84 m; Table 1 ), which means that rainwater would dilute in a few tenths of metres during formation of that warm water mass. Indeed, lignin-derived phenols, highly modified by photo-oxidation, have been found in dissolved and submicron particles suspended in the North Pacific Subtropical Mode Water, suggesting an aerosol source for these fluorescent materials [27] . The high archetypal tyrosine-like fluorescence (C4) of the aged Central waters (AOU>200 μmol kg −1 ) of the Equatorial (13EqPac) and Central North Pacific (CMW NP ) might be due also to both WT that occupy shallow layers (archetypal depths 253±13 m for CMW NP and 483±35 m for 13EqPac; Table 1 ), where protein-like fluorescence is higher because of the proximity to the epipelagic waters, where these materials are usually produced [6] . The turnover times of the fluorescent materials (timescale of centuries) are of the same order of magnitude of the turnover time of the bulk DOC [11] , but an order of magnitude faster than the apparent age of the ocean DOC as derived from 14 C measurements (timescale of millennia) [2] . However, it should be noted that mean age, derived from 14 C involved by nuclear tests, is not homologous with turnover time (mean transit time), derived from total reservoir and fluxes entering/leaving the reservoir. It is remarkable that the observed decrease in the tyrosine-like fluorescence in the dark ocean is at centennial timescales. It has been reported that the turnover of these fluorophores in the surface ocean is on a timescale of days [6] , [28] , but this long-term decline in tyrosine-like fluorescence in the dark global ocean, coupled to water mass ageing, has never been reported. We can hypothesize that a minor fraction of the tyrosine-like fluorescence is processed on the scale of centuries, whereas the bulk of the signal has a turnover time on the order of days to weeks. Furthermore, this apparent discrepancy could also be related to the different turnover of the set of compounds that are represented by this fluorescence signature [29] . We conclude that humic-like fluorescence (C1 and C2) reveals a suitable marker of the production of optically active RDOM with turnover times of 400–600 years. Using the oceans as an incubator, our measurements indicate that the in situ microbial production of fluorescent humic-like materials in the dark global ocean is a sink of reduced carbon in the timescale of hundreds of years. Conversely, the turnover time of the tyrosine-like component (C4) was compatible with the turnover time of the bulk DOC and both decline with water mass ageing. This coincidence between the turnover times of the bulk DOC pool and the tyrosine-like component could also have applications for tracing long-term DOC reactivity in the dark ocean. Sample collection A total of 147 stations were sampled from 40°S to 34°N in the Atlantic, Indian and Pacific Oceans (Malaspina 2010 Expedition, from December 2010 to July 2011). Vertical profiles of salinity ( S ), potential temperature ( θ ) and dissolved oxygen (O 2 μmol kg −1 ) were recorded continuously with the conductivity–temperature–depth (CTD) and oxygen sensors installed in the rosette sampler. Salinity and dissolved oxygen were calibrated against bottle samples determined on board with a salinometer and the Winkler method, respectively. The AOU was calculated as the difference between the saturation and measured dissolved oxygen. Oxygen saturation was calculated from salinity and potential temperature [30] . Bottle depths were chosen on the basis of the CTD-O 2 profiles to cover as much water masses as possible of the dark global ocean. Seawater samples for fluorescence measurements, collected in 12 l Niskin bottles, were immediately poured into glass bottles and stored in dark conditions until measurement within 6 h from collection. We collected 800 water samples from 200 to 4,000 m depth. Fluorescence spectral acquisition When the coloured fraction of marine DOM (CDOM) is irradiated with ultraviolet light, it emits a fluorescence signal characteristic of both amino-acid- and humic-like compounds, which is collectively termed FDOM [10] . Fluorescence excitation–emission matrices (EEMs) were collected with a JY-Horiba Spex Fluoromax-4 spectrofluorometer at room temperature (around 20 °C) using 5 nm excitation and emission slit widths, an integration time of 0.25 s, an excitation range of 240–450 nm at 10 nm increments and an emission range of 300–560 nm at 2 nm increments. To correct for lamp spectral properties and to compare results with those reported in other studies, spectra were collected in signal-to-reference (S:R) mode with instrument-specific excitation and emission corrections applied during collection, and EEMs were normalized to the Raman area (RA). In our case, the RA and its baseline correction were performed with the emission scan at 350 nm of the Milli-Q water blanks and the area was calculated following the trapezoidal rule of integration [29] . To track the variability of the instrument in the Raman, protein- and humic-like regions of the spectrum during the 147 working days of the expedition and assess gradual spectral bias, three standards were run daily: (1) a P-terphenyl block (Stranna) that fluoresces in the protein region, between 310 and 600 nm exciting at 295 nm; (2) a tetraphenyl butadiene block (Stranna) that fluoresces in the humic region, between 365 and 600 nm exciting at 348 nm; and (3) a sealed Milli-Q cuvette (Perkin Elmer) scanned between 365 and 450 nm exciting at 350 nm. Supplementary Figure 1a shows that the temporal evolution of the RA of the Milli-Q water used on board and the reference P-terphenyl and tetraphenyl butadiene materials were parallel, which confirms that the Raman normalization was successful in both the protein- and the humic-like regions of the EEMs. Therefore, no additional drift corrections were necessary. The comparison between the reference sealed Milli-Q (sMQ) and the daily Milli-Q water allowed us to demonstrate that the Milli-Q water used on board was of a good quality ( Supplementary Fig. 1b ). The average coefficient of variation between the sMQ and Milli-Q water throughout the circumnavigation was only 0.81%. Similarly, two scans of the reference sealed Milli-Q were measured at the beginning (sMQ 1 ) and at the end (sMQ 2 ) of each session, which reveals a slight shift of the fluorescence intensities along each working day ( Supplementary Fig. 1c ). The initial and final sMQ spectra were separated by about 10 h of continuous work of the spectrofluorometer. We found that the average coefficient of variation between sMQ 1 and sMQ 2 was 1.62%. Therefore, the daily instrument shift was low and about twice the long-term variability throughout the circumnavigation. Inner-filter correction was not applied due to the low absorption coefficient of CDOM of the samples collected during the circumnavigation: 1.01±0.04 m −1 (average±s.d.) at 250 nm, that is, much lower than the threshold of 10 m −1 above which this correction is required [8] . Raman-normalized Milli-Q blanks were subtracted to remove the Raman scattering signal [31] , [32] . RA normalization, blank subtraction and generation of EEMs were performed using MATLAB (version R2008a). Global PARAFAC modelling PARAFAC was used to identify the fluorescent components that comprise the EEMs in the global ocean. PARAFAC was performed using the DOMFluor 1_7 Toolbox [8] . Before the analysis, Rayleigh scatter bands (first order at each wavelength pair where Ex=Em±bandwidth; second order at each wavelength pair where Em=2 × Ex±(2 × bandwidth)) were trimmed. The global PARAFAC model was derived based on 1,574 corrected EEMs and was validated using split-half validation and random initialization [8] . A four-component model was obtained ( Supplementary Fig. 2 ), two of them of humic-like nature, peak A/C (at Ex/Em <270–370/470 nm) and peak M (at Ex/Em 320/400 nm), and two of amino-acid-like nature, attributed to tryptophan and tyrosine at 290/340 and 270/310 nm [8] , respectively. Here we report the maximum fluorescence ( F max) in Raman units (RU) (refs. 31 , 32 ). Multi-parameter water mass analysis The dark ocean (from 200 m to the bottom) can be described by the mixing of prescribed WT, characterized by a unique combination of thermohaline and chemical property values. Water mass analysis quantifies the proportions of the WT that contribute to a given water sample. In our case, we have characterized the WT on the basis of its salinity ( S ) and potential temperature ( θ ), which are assumed to be conservative parameters and, therefore, they do not change from the area where the WT are defined to the study area. The equations to be solved for a water sample j are: where x ij is the proportion of WT i in sample j; θ j and S j are the thermohaline characteristics of sample j; and θ i and S i are the prescribed thermohaline characteristics of WT i in the area where it is defined. Furthermore, the solution of the multi-parameter water mass analysis includes an additional constraint, that is, all contributions ( x ij ) have to be non-negative. We identified 18 water masses and 22 WT on the route sampled and their characteristics are summarized in Supplementary Table 1 . They were divided into three domains according to their depth: central, intermediate and abyssal waters. In the central domain, there are Eighteen Degrees Water (EDW), Eastern North Atlantic Central Water (ENACW), defined by two WT of 12 and 15 °C, Equatorial Atlantic Central Water (13 °C; 13EqAtl), South Atlantic Central Water (SACW), defined by two WT of 12 and 18 °C, Indian Subtropical Mode Water (STMW I ), Indian Central Water (13 °C; ICW 13 ), South Pacific Subtropical Mode Water (STMW SP ), South Pacific Central Water (20 °C; SPCW 20 ), Equatorial Pacific Central Water (13 °C; 13EqPac), North Pacific Subtropical Mode Water (STMW NP ) and North Pacific Central Mode Water (12 °C; CMW NP ). In the intermediate domain, we found Mediterranean Water (MW), Sub-Antarctic Mode Water (SAMW), Antarctic Intermediate Water (AAIW), defined by two WT of 3.1 and 5.0 °C, and North Pacific Intermediate Water (NPIW). In the abyssal domain, there are Circumpolar Deep Water (1.6 °C; CDW), North Atlantic Deep Water (NADW), defined by two types of 2 and 4.6 °C, and Antarctic Bottom Water (AABW). Equations (1)–(3), ,  can be solved for a maximum of three WT simultaneously. Given that we have identified 22 WT, we have grouped the WT in the triads presented in Supplementary Table 2 on the basis of reasonable vertical and geographical constraints to the water mass mixing usually applied in the analysis of water masses. Concerning the vertical constraints, for a given region of the ocean, every WT will mix only with the WT situated immediately above and below according to their density. Concerning the geographical constraints, every WT will mix preferentially with WT in their surroundings. The multi-parameter water mass analysis was applied to the 800 samples from the dark ocean ( θ <18 °C, AOU>0) where corresponding measurements of fluorescence ( F max1, F max2, F max3 and F max4) and AOU were obtained. Once the WT proportions ( x ij ) are known, the proportion of the total volume of water sampled that corresponds to WT i (%VOL i ) can be calculated as: Where n =800 is the number of deep samples. Archetypal values of F max and AOU for each WT Using the measured values of fluorescence and AOU ( N ) and the proportions of the 22 WT identified in this study ( x ij ), the water mass proportion-weighted average concentration of N in each WT, N i , termed archetypal value of N , can be calculated as [12] : where N j is the concentration of N in sample j. The s.d. of the estimated archetypal value of N i was obtained by: Similarly, the archetypal value of variable N in every sample ( N j ) was calculated as follows: The determination coefficient ( R 2 ) and the s.d. of the residual (s.d. res) of the linear regressions of N j (measured values) versus < N j > (archetypal values) allows assessing the degree of dependence of variable N on WT mixing in the dark ocean. Application of equations (5) and (6) to the collection depth of the samples ( Z i ) allows obtaining the archetypal depth of each WT ( Z i ) and its corresponding s.d. ( Z i ). NFP and turnover times of the components The tight relationship between fluorescence intensity and AOU for components C1, C2 and C4 allows estimating the rate of change of F max per AOU unit (∂ F max/∂AOU). It was calculated as the first derivative of the power functions fitting F max i and AOU i ( Fig. 4 ). Then, the global net production of each fluorescence component, NFP (in RU per year), was calculated as: where is the WT proportion-weighted fluorescence change rate per AOU unit of the global dark ocean. The OCR was calculated by dividing 0.827 pmol O 2 per year, a conservative estimate of the global oxygen demand of the dark ocean based on organic carbon sedimentation fluxes [16] , by 1.38 × 10 21 kg, which is the mass of the ocean at a depth >200 m. Once the NFP of the three components was obtained, we calculated their respective turnover time ( τ ): Where is the WT proportion-weighted average fluorescence of the dark global ocean. How to cite this article : Catalá, T. S. et al. Turnover time of fluorescent dissolved organic matter in the dark global ocean. Nat. Commun. 6:5986 doi: 10.1038/ncomms6986 (2015).